Plasticity and redundancy among AMA–RON pairs ensure host cell entry ofToxoplasmaparasites Malaria and toxoplasmosis are infectious diseases caused by the apicomplexan parasites Plasmodium and Toxoplasma gondii , respectively. These parasites have developed an invasion mechanism involving the formation of a moving junction (MJ) that anchors the parasite to the host cell and forms a ring through which the parasite penetrates. The composition and the assembly of the MJ, and in particular the presence of protein AMA1 and its interaction with protein RON2 at the MJ, have been the subject of intense controversy. Here, using reverse genetics, we show that AMA1, a vaccine candidate, interacts with RON2 to maintain the MJ structural integrity in T. gondii and is subsequently required for parasite internalization. Moreover, we show that disruption of the AMA1 gene results in upregulation of AMA1 and RON2 homologues that cooperate to support residual invasion. Our study highlights a considerable complexity and molecular plasticity in the architecture of the MJ. Key members of the phylum Apicomplexa include Plasmodium spp. and Toxoplasma gondii , which are the causative agents of malaria and toxoplasmosis, respectively. These protozoans are obligate intracellular parasites that share a unique, multi-step invasion mechanism. Initially, a ‘distant’ attachment is mediated by proteins secreted from the micronemes (MICs) and targeted to the parasite cell surface where they engage host cell receptors [1] . This step triggers subsequent secretion of the rhoptries [2] and the formation of an electron-dense layer referred to as the moving junction (MJ) that demarcates the closely apposed parasite and host cell membranes [3] . Formation of the MJ is considered as the irreversible attachment step necessary for a successful invasion. The parasite then actively passes through the MJ, apparently using an actin–myosin motor [4] , resulting in complete encapsulation of the parasite into the parasitophorous vacuole membrane (PVM). Assembly of the MJ relies on the export of a complex of four rhoptry neck proteins (RON2, RON4, RON5 and RON8) into the host cell where RON2 is integrated into the host plasma membrane with its N-terminal domain directed into the host cytosol, where it is likely retaining RONs 4, 5 and 8 to the cytosolic face of the host membrane [5] , [6] . The identities of proteins presented at the parasite cell surface that contribute to the MJ, however, remain a matter of debates [7] , [8] , [9] . At the core of this controversy, the transmembrane apical membrane antigen 1 (AMA1), a MIC protein that relocalizes to the entire surface of the parasite before invasion, has been shown to form part of the RON complex in vitro [5] , [10] . AMA1 interacts directly with the extracellular C-terminal portion of RON2 (refs 5 , 6 , 11 ) and through substantial induced fit forms a high-affinity complex [12] , [13] . Molecules interfering with AMA1–RON2 interaction severely block invasion both in T. gondii and in Plasmodium falciparum [6] , [11] , [14] , supporting a model whereby the AMA1–RON2 complex forms the intimate contact between the parasite and host plasma membranes. This model, however, does not capture whether this complex constitutes the primary site of traction used by the parasites to invade the host cell. Despite the breadth of data supporting the role of AMA1 in assembling the MJ [6] , [11] , [12] , [13] , [14] , [15] , [16] , [17] , recent studies question a critical role of AMA1–RON2 interaction in MJ formation. AMA1 is instead considered as most MICs to function in an earlier recognition/attachment step preceding MJ formation [8] , [9] . These conclusions are largely based on the observations that the AMA1 gene is dispensable and that AMA1-deficient (TgAMA1 KO ) T. gondii are impaired in host cell attachment but displayed internalization with normal kinetics through a MJ labelled with RON2 or RON4 (ref. 8 ). This recent model excludes the possibility of a compensatory mechanism for MJ formation and, importantly, does not consider the possibility that failure to establish a firm junction would lead to parasite detachment from the host cell. Here we show that point mutations in a loop present in TgRON2 specifically impair AMA1 binding and disrupt MJ formation, thereby demonstrating that AMA1 and RON2 cooperate to shape the MJ. We also demonstrate that once the MJ is formed, the cytoplasmic tail of AMA1 participates in the internalization step. Finally, we generate a TgAMA1-null cell line (KO-AMA1) and reveal that its residual invasion is ensured by (i) an AMA1-like protein (AMA2) that is functionally redundant by coordinating RON2 and structuring the MJ; and possibly by (ii) a newly identified RON–AMA homologue pair (RON2 L1 –AMA4). This study highlights considerable genetic and molecular plasticity of the T. gondii genome to compensate for dysfunction in the core MJ machinery. Furthermore, we reveal a complex architecture of the MJ that comprises evolutionary divergent AMA–RON pairs. Depletion of RON2 leads to a severe invasion defect The role of RON2 in MJ formation has never been investigated by genetic approaches. Here we generated a conditional knockdown T. gondii cell line for RON2 , named KD-RON2 for knockdown RON2, by replacing the endogenous promoter with an anhydrotetracycline (ATc)-repressible promoter ( Fig. 1a and Supplementary Fig. 1a ). No signal was detected by using western blot or by immunofluorescence assay (IFA) in the neck using anti-RON2 antibodies, even in the absence of ATc ( Fig. 1b,c ), showing that expressing the RON2 gene under the control of an inducible promoter is detrimental to correct expression, timing and protein stability. The plaque assay, which recapitulates all the steps of the lytic cycle, revealed that RON2 is critical for parasite survival ( Fig. 1d ). The KD-RON2 cell line formed very small plaques as compared with the parental strain, even in the absence of ATc. Although intracellular growth was not primarily affected ( Supplementary Fig. 1b ), a severe block in host cell invasion down to 10% that of the control strain was observed ( Fig. 1e ). This defect could be largely restored by complementation of the mutant with a wild-type copy of the RON2 gene (see Supplementary Fig. 2 for genetic and phenotypic characterizations of the complemented KD-RON2 lines). 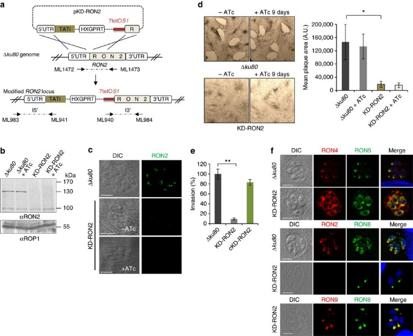Figure 1: Isolation and phenotypic characterization of KD-RON2 parasites. (a) Scheme illustrating the approach used to generate a conditional knockout of theRON2gene. TheRON25′UTR was cloned upstream of the transactivator TATi, while the 5′ coding sequence ofRON2was cloned downstream of the inducible 7tetOS1 promoter. TheHXGPRT(hypoxanthine xanthine guanine phosphoribosyl transferase) gene was used to select for pKD-RON2 plasmid inT. gondii. The recombination at theRON2locus by double-homologous recombination was verified with PCRs I5′, I3′ andRON2, using primer pairs ML983/ML941, ML940/ML984 and ML1472/ML1473, respectively (seeSupplementary Table 2for primer sequences). (b) Immunoblot of RON2 in Δku80and KD-RON2 strains previously grown in ±ATc for 8 days. ROP1, loading control. (c) IFA of Δku80or KD-RON2 parasites previously grown for 3 days with ±ATc using anti-RON2-4 antibodies. DIC: Differential Interference Contrast. Scale bars, 5 μm. (d) Plaque assays of HFFs monolayers infected with either parental (Δku80) or KD-RON2 lines pre-treated or not during 2 days with ATc and grown with ATc for the next 7 days. Quantification of the size of the lysis plaques is shown in the graph. Student’st-test, *P<0.05; mean±s.e.m (n=3). (e) Invasion assay for 30 min of Δku80, KD-RON2 and complemented KD-RON2 (cKD-RON2) lines. Student’st-test, **P<0.01; mean±s.e.m (n=3). (f) IFA of RON2, RON4, RON5, RON8 and RON9 in intracellular Δku80or KD-RON2 parasites grown without ATc. Scale bars, 5 μm. Figure 1: Isolation and phenotypic characterization of KD-RON2 parasites. ( a ) Scheme illustrating the approach used to generate a conditional knockout of the RON2 gene. The RON2 5′UTR was cloned upstream of the transactivator TATi, while the 5′ coding sequence of RON2 was cloned downstream of the inducible 7tetOS1 promoter. The HXGPRT (hypoxanthine xanthine guanine phosphoribosyl transferase) gene was used to select for pKD-RON2 plasmid in T. gondii . 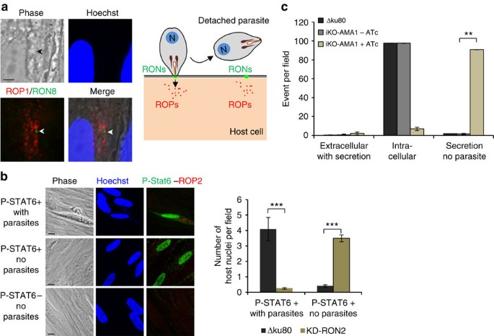Figure 2: Both AMA1 and RON2 are crucial for MJ formation. (a) IFAs of KD-RON2 mutant following a 5-min invasion assay revealing clusters of ROP1-positive vesicles associated with a dot of RON8 (white arrow) in the host cells despite the absence of attached parasite (black arrow). The nuclei of the host cell were stained with Hoechst. Schematic illustrating the abortive invasions is shown in the right panel. (b) Failure of MJ formation monitored by a phospho-STAT6 assay. The injection of ROPs proteins in the host cell by Δku80or KD-RON2 cell lines was quantified following IFA using anti-ROP2-3-4 to visualize the parasites vacuoles and anti-P-STAT6 to label the host cell nuclei following ROP16-induced nuclear translocation of phospho-STAT6. The nuclei were also stained with Hoechst. Non-infected HFFs were used as a control (P-STAT6−, no parasites). Scale bars, 5 μm. Student’st-test, ***P<0.001; mean±s.e.m. (n=3). (c) Quantification of productive and abortive invasions in the parental Δku80and inducible knockdown AMA1 cell lines treated with ±ATc. The number of intracellular parasites and ROP1 vesicles containing a RON4 dot without any parasite (abortive invasion) were counted following IFA using anti-ROP1 and anti-RON4 4H1. Student’st-test, **P<0.01; mean±s.e.m. (n=3). The recombination at the RON2 locus by double-homologous recombination was verified with PCRs I5′, I3′ and RON2 , using primer pairs ML983/ML941, ML940/ML984 and ML1472/ML1473, respectively (see Supplementary Table 2 for primer sequences). ( b ) Immunoblot of RON2 in Δ ku80 and KD-RON2 strains previously grown in ±ATc for 8 days. ROP1, loading control. ( c ) IFA of Δ ku80 or KD-RON2 parasites previously grown for 3 days with ±ATc using anti-RON2-4 antibodies. DIC: Differential Interference Contrast. Scale bars, 5 μm. ( d ) Plaque assays of HFFs monolayers infected with either parental (Δ ku80 ) or KD-RON2 lines pre-treated or not during 2 days with ATc and grown with ATc for the next 7 days. Quantification of the size of the lysis plaques is shown in the graph. Student’s t -test, * P <0.05; mean±s.e.m ( n =3). ( e ) Invasion assay for 30 min of Δ ku80 , KD-RON2 and complemented KD-RON2 (cKD-RON2) lines. Student’s t -test, ** P <0.01; mean±s.e.m ( n =3). ( f ) IFA of RON2, RON4, RON5, RON8 and RON9 in intracellular Δ ku80 or KD-RON2 parasites grown without ATc. Scale bars, 5 μm. Full size image We then investigated the expression and cellular location of the other members of the junctional complex in the KD-RON2 parasites. RON4 and RON5 were not properly expressed ( Supplementary Fig. 1d ) and localized within parasite cells in absence of RON2. They were not associated with the rhoptry neck, but instead staining was observed in the parasitophorous vacuole (PV) or perinuclear ( Fig. 1f ). Consequently, RON4 and RON5 were not detected outside the parasite during invasion ( Supplementary Fig. 1c ). Surprisingly, RON8 correctly localized to the rhoptries ( Fig. 1f ), and more importantly was found associated with the MJ during invasion in the KD-RON2 parasites that could successfully invade ( Supplementary Fig. 1c ), indicating that a MJ was formed during invasion of the KD-RON2 parasites. Collectively, these results demonstrate the critical role of RON2 during invasion and suggest that additional components can associate with RON8 to form the MJ. AMA1 and RON2 mutants are impaired in MJ formation Following invasion by KD-RON2 parasites, we observed the presence of clusters of vesicles labelled with rhoptry marker ROP1 inside the host cell, associated with a dot of RON8, although no parasite could be observed in the vicinity ( Fig. 2a ). This particular event corresponds to the secretion of rhoptry content into the host cell and proves that the mutant successfully completed the initial step of attachment and initiated a MJ, although it failed to invade and eventually detached. In consequence, these ROP1 ‘clouds’ reflect unsuccessful MJ-dependent intimate attachment. We then quantified these abortive invasion events using an assay based on the injection of the rhoptry kinase ROP16 into the host that causes rapid phosphorylation and nucleus translocation of STAT6 (ref. 18 ). The non-infected cells that were phospho-STAT6-positive (P-STAT6 + ) reflect the abortive invasion following rhoptry secretion. The percentage of P-STAT6 + cells in the absence of intracellular parasites was substantially increased in the KD-RON2 parasites compared with the Δ ku80 parental line ( Fig. 2b ). Coincidentally, the inducible AMA1 knockout line (iKO-AMA1) [19] revealed the same abnormal detachment following the depletion of AMA1 ( Fig. 2c ). In conclusion, depletion of either AMA1 or RON2 compromises the capacity of the parasite to establish a robust intimate attachment with the host cell. Figure 2: Both AMA1 and RON2 are crucial for MJ formation. ( a ) IFAs of KD-RON2 mutant following a 5-min invasion assay revealing clusters of ROP1-positive vesicles associated with a dot of RON8 (white arrow) in the host cells despite the absence of attached parasite (black arrow). The nuclei of the host cell were stained with Hoechst. Schematic illustrating the abortive invasions is shown in the right panel. ( b ) Failure of MJ formation monitored by a phospho-STAT6 assay. The injection of ROPs proteins in the host cell by Δ ku80 or KD-RON2 cell lines was quantified following IFA using anti-ROP2-3-4 to visualize the parasites vacuoles and anti-P-STAT6 to label the host cell nuclei following ROP16-induced nuclear translocation of phospho-STAT6. The nuclei were also stained with Hoechst. Non-infected HFFs were used as a control (P-STAT6−, no parasites). Scale bars, 5 μm. Student’s t -test, *** P <0.001; mean±s.e.m. ( n =3). ( c ) Quantification of productive and abortive invasions in the parental Δ ku80 and inducible knockdown AMA1 cell lines treated with ±ATc. The number of intracellular parasites and ROP1 vesicles containing a RON4 dot without any parasite (abortive invasion) were counted following IFA using anti-ROP1 and anti-RON4 4H1. Student’s t -test, ** P <0.01; mean±s.e.m. ( n =3). Full size image AMA1–RON2 pair establishes the MJ To date, the functional evidence in support of a role for the AMA1–RON2 interaction in MJ formation is based on the inhibition of parasite invasion by antibodies or peptides that prevent the complex formation in vitro [6] , [11] , [12] , [13] , [14] , [15] , [16] , [17] . To test these observations, we produced a RON2 mutant selectively compromised in AMA1 binding by complementation of the KD-RON2 with a copy of RON2 that was either wild-type or mutated at residues I 1318 and L 1319 (RON2 WT and RON2 IL/AA , respectively; Supplementary Fig. 2 ); these residues have been previously shown in vitro to be important for AMA1 binding [12] . Both RON2 WT and RON2 IL/AA were expressed at comparable levels ( Fig. 3a and Supplementary Fig. 2c ), localized to the neck of the rhoptries and restored both the proper trafficking of the whole complex to the rhoptries ( Fig. 3b ) and its translocation at the MJ ( Supplementary Fig. 2d ). Importantly, a marked decrease in the capacity of AMA1 to co-immunopurify RON2 was observed in the RON2 IL/AA compared with RON2 WT ( Fig. 3c ) that correlated with a significant defect in invasion ( Fig. 3d ). Consistent with a cooperative role of AMA1–RON2 in assembling the MJ, we also showed a substantial abortive invasion in the RON2 IL/AA line ( Fig. 3e ) or by incubating the Δ ku80 parental line with a RON2 peptide competing for the AMA1–RON2 interaction (TgRON2sp) [12] ( Fig. 3f ). 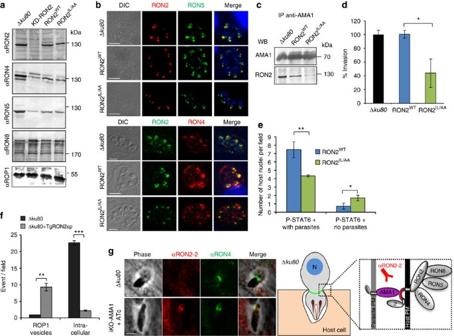Figure 3: AMA1 and RON2 interact at the MJ to intimately attach the parasite to the host cell. (a) Immunoblots or (b) IFA of RON2, RON4, RON5 and RON8 on Δku80, KD-RON2 or complemented RON2WTand RON2IL/AAcell lines. ROP1, loading control. DIC: Differential Interference Contrast. Scale bars, 5 μm. (c) Western blot (WB) of a co-immunoprecipitation using anti-AMA1 antibodies on Δku80, cKD-RON2 WT and cKD-RON2 IL/AA lysates, and further revealed with anti-AMA1 or anti-RON2 antibodies. (d) Invasion assay performed for 5 min using Δku80, complemented RON2WTand RON2IL/AAparasites. Dual labelling with anti-SAG1 and anti-ROP1 antibodies was used to discriminate between extra- and intracellular parasites. Student’st-test, *P<0.05; mean±s.e.m. (n=3). (e) Quantification of abortive invasions in complemented RON2WTand RON2IL/AAusing P-STAT6 assay. Student’st-test, **P<0.01, *P<0.05; mean±s.e.m. (n=3). (f) Quantification of productive and abortive invasions in Δku80line incubated with ±5 μM synthetic TgRON2 peptide (TgRON2sp). ‘Events’ refer to either ROP1 vesicles or intracellular parasites. The numbers of intracellular parasites identified as PVM-associated ROP1 labelling, and ROP1 vesicles containing a RON4 dot without any parasite were quantified following IFA. Student’st-test, **P<0.01, ***P<0.001; mean±s.e.m. (n=3). (g) Left, IFAs performed on invading Δku80or ATc-treated iKO-AMA1 parasites using anti-RON2-2 antibodies directed against the AMA1-binding domain of RON2. Right, scheme depicting the MJ organization; PM, plasma membrane; red, AMA1-binding domain of RON2 recognized by anti-RON2-2. Figure 3: AMA1 and RON2 interact at the MJ to intimately attach the parasite to the host cell. ( a ) Immunoblots or ( b ) IFA of RON2, RON4, RON5 and RON8 on Δ ku80 , KD-RON2 or complemented RON2 WT and RON2 IL/AA cell lines. ROP1, loading control. DIC: Differential Interference Contrast. Scale bars, 5 μm. ( c ) Western blot (WB) of a co-immunoprecipitation using anti-AMA1 antibodies on Δ ku80 , cKD-RON2 WT and cKD-RON2 IL/AA lysates, and further revealed with anti-AMA1 or anti-RON2 antibodies. ( d ) Invasion assay performed for 5 min using Δ ku80 , complemented RON2 WT and RON2 IL/AA parasites. Dual labelling with anti-SAG1 and anti-ROP1 antibodies was used to discriminate between extra- and intracellular parasites. Student’s t -test, * P <0.05; mean±s.e.m. ( n =3). ( e ) Quantification of abortive invasions in complemented RON2 WT and RON2 IL/AA using P-STAT6 assay. Student’s t -test, ** P <0.01, * P <0.05; mean±s.e.m. ( n =3). ( f ) Quantification of productive and abortive invasions in Δ ku80 line incubated with ±5 μM synthetic TgRON2 peptide (TgRON2sp). ‘Events’ refer to either ROP1 vesicles or intracellular parasites. The numbers of intracellular parasites identified as PVM-associated ROP1 labelling, and ROP1 vesicles containing a RON4 dot without any parasite were quantified following IFA. Student’s t -test, ** P <0.01, *** P <0.001; mean±s.e.m. ( n =3). ( g ) Left, IFAs performed on invading Δ ku80 or ATc-treated iKO-AMA1 parasites using anti-RON2-2 antibodies directed against the AMA1-binding domain of RON2. Right, scheme depicting the MJ organization; PM, plasma membrane; red, AMA1-binding domain of RON2 recognized by anti-RON2-2. Full size image Finally, using antibodies directed against the AMA1-binding site of RON2 (ref. 5 ) (see scheme on Fig. 3g ), we showed that this site was inaccessible to immunostaining when AMA1 is expressed, while in most of the iKO-AMA1 parasites depleted in AMA1 the constriction displayed labelling ( Fig. 3g ). These results establish the existence of an embedded interaction between AMA1 and RON2 at the MJ, and reveal a different organization of the MJ in absence of AMA1. Altogether, these results demonstrate that the binding of RON2 to AMA1 is responsible for the structural integrity of the MJ required to efficiently proceed further in the invasion process. AMA1 is involved in parasite internalization Previous studies have reported the importance of the AMA1 cytoplasmic tail in invasion by both T. gondii and P. falciparum [20] , [21] . In Toxoplasma , the expression of a copy of AMA1 with mutations in the cytoplasmic domain (AMA1 FW/AA ) does not rescue the invasion defect of the iKO-AMA1 in the presence of ATc [20] . However, whether the AMA1 tail functions as sensing device triggering rhoptry secretion, MJ formation or parasite internalization has not been further investigated. Here we dissected these steps by IFA ( Fig. 4 ). In contrast to abortive invasions observed previously with the iKO-AMA1 following ATc treatment, the AMA1 FW/AA parasites remain attached through a MJ but failed to proceed further in internalization ( Fig. 4a,b ). This feature is reminiscent of cytochalasin-treated tachyzoites that discharge rhoptries, attach to host cell, form a MJ, but cannot penetrate ( Fig. 4c ) [22] , [23] . This result demonstrates for the first time that following its interaction with RON2 and MJ formation, AMA1 is necessary for subsequent internalization of the parasite. These data also highlight once more the structural role of the AMA1–RON2 interaction, as the functional ecotodomain of AMA1 FW/AA stabilizes the intimate attachment to the host via its binding to RON2, thus preventing disengagement. Taken together, these findings reveal the dual role of AMA1 in MJ formation and internalization. 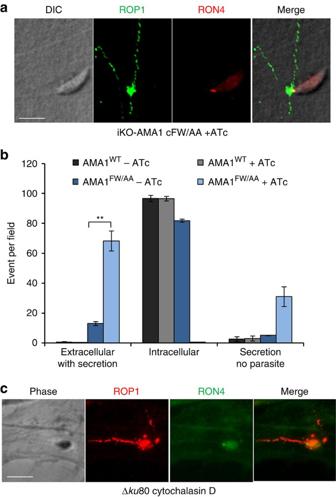Figure 4: The AMA1 tail functions as a downstream signal for internalization. (a) IFAs of invasion assay carried out on ATc-treated iKO-AMA1 cFW/AA (iKO-AMA1 complemented with AMA1FW/AA); green, ROP1-positive vesicles; red, MJ labelled with RON4. DIC: Differential Interference Contrast. Scale bar, 5 μm. (b) Quantification of the numbers of attached extracellular parasites with a MJ formed, intracellular parasites and abortive invasion for AMA1WT(iKO-AMA1 complemented with wild-type AMA1) or AMA1FW/AAfollowing IFAs described ina. Student’st-test, **P<0.01; mean±s.e.m. (n=3). (c) IFA of Δku80following invasion assay in presence of cytochalasin D. Evacuoles are labelled with anti-ROP1 and the MJ is detected by anti-RON4 Mab T5 4H1. Scale bar, 5 μm. Figure 4: The AMA1 tail functions as a downstream signal for internalization. ( a ) IFAs of invasion assay carried out on ATc-treated iKO-AMA1 cFW/AA (iKO-AMA1 complemented with AMA1 FW/AA ); green, ROP1-positive vesicles; red, MJ labelled with RON4. DIC: Differential Interference Contrast. Scale bar, 5 μm. ( b ) Quantification of the numbers of attached extracellular parasites with a MJ formed, intracellular parasites and abortive invasion for AMA1 WT (iKO-AMA1 complemented with wild-type AMA1) or AMA1 FW/AA following IFAs described in a . Student’s t -test, ** P <0.01; mean±s.e.m. ( n =3). ( c ) IFA of Δ ku80 following invasion assay in presence of cytochalasin D. Evacuoles are labelled with anti-ROP1 and the MJ is detected by anti-RON4 Mab T5 4H1. Scale bar, 5 μm. Full size image RON2 can engage an AMA1-homologue protein To decipher the architecture of the MJ in complete absence of AMA1, we generated an AMA1 null strain (KO-AMA1) using a gene disruption strategy by single homologous recombination ( Fig. 5a and Supplementary Fig. 3a ). Following vector integration, a truncated version of AMA1 containing only the first 184 residues (~20 kDa) might be expressed, but importantly this interrupted copy does not contain the functional RON2-binding domain. A clone was isolated following a 2-month selection process that was AMA1 negative by IFA and western blot ( Fig. 5b,c ). Although the mutant replicated at a similar rate to the parental line ( Supplementary Fig. 3b ), a severe defect in invasion was observed with an invasion efficiency reduced by 90% compared with the parental line ( Fig. 5d ). Similar to the conditional iKO-AMA1, KO-AMA1 parasites were impaired in MJ formation ( Fig. 5e ), although the remaining invaders displayed a characteristic ring-shape RON signal at the interface of the host–parasite plasma membranes ( Supplementary Fig. 3c ), clearly establishing that AMA1 is not involved in the targeting of the RON2/RON4/RON5/RON8 complex at the MJ, and that the parasite can successfully invade by a MJ-dependent process in the absence of AMA1. Importantly, the invasion rate of KO-AMA1 increased in continuous culture to reach 20% after 12 months, suggesting that the mutant is capable of moderate adaptation to bypass the deleterious AMA1 inactivation ( Fig. 5d ). The potential for a compensatory mechanism was further supported by an in situ binding assay [6] , indicating that RON2 binds to an additional MIC protein to promote invasion. Indeed, a recombinant GST fusion protein of the AMA1-binding domain of RON2 (GST-RON2-2) or the synthetic peptide TgRON2sp [12] still recognized a MIC protein in the KO-AMA1 mutant ( Fig. 5f ) and exhibited an invasion inhibitory effect ( Fig. 5g ). It has to be noted that neither GST-RON2-2 labelling nor significant inhibition of invasion were previously detected in the mutant when assayed just after the clone isolation, i.e., 2 months following transfection. This tends to suggest that this hypothetical partner had been upregulated over time to compensate for the loss of AMA1. 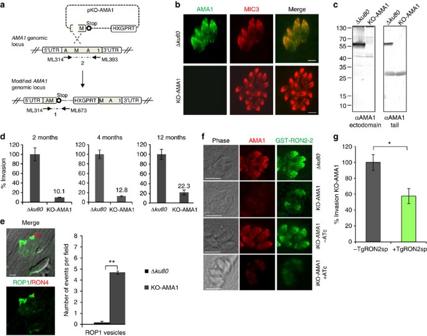Figure 5: Adaptation of KO-AMA1 parasites to partially compensate the loss of AMA1. (a) Scheme depicting theAMA1disruption strategy by single homologous recombination. An internal fragment of theAMA1gene was cloned in the p3Ty-HXGPRT vector, giving pKO-AMA1. This vector contains theHXGPRTgene (hypoxanthine xanthine guanine phosphoribosyl transferase) for plasmid selection inT. gondii.Vector integration in Δku80genome was verified with PCRs 1 and 2 using the primer pairs ML314/ML673 and ML314/ML393, respectively (seeSupplementary Table 2for primer sequences), and led to the disruption ofAMA1in two non-functional copies. (b) IFAs on intracellular Δku80or KO-AMA1 strains using anti-AMA1 ectodomain and anti-MIC3 antibodies. Scale bars, 5 μm. (c) Immunoblot carried out on Δku80or KO-AMA1 parasites shows the absence of AMA1 in the mutant using anti-AMA1 antibodies directed against the full ectodomain (domains DI, DII and DIII) and anti-AMA1 tail antibodies. (d) Invasion rates of Δku80and KO-AMA1 compared over time during a 5-min invasion assay. Intracellular parasites were scored using a red–green differential antibody staining. Values represent mean±s.e.m (n=3). (e) Left panel: IFAs of KO-AMA1 parasites following invasion assay; red arrow, rhoptry secretion in absence of attached parasite. Scale bar, 5 μm. Right panel: quantification of the abortive invasions in Δku80and KO-AMA1 cell lines. Student’st-test, **P<0.05; mean±s.e.m. (n=3). (f)In situhybridization assay in KO-AMA1 using GST-RON2-2 protein reveals an additional MIC partner for RON2, different from AMA1. Scale bars, 5 μm. (g) Invasion rates of KO-AMA1 parasites ±5 μM TgRON2sp. Student’st-test, *P<0.05; mean±s.e.m. (n=3). Figure 5: Adaptation of KO-AMA1 parasites to partially compensate the loss of AMA1. ( a ) Scheme depicting the AMA1 disruption strategy by single homologous recombination. An internal fragment of the AMA1 gene was cloned in the p3Ty-HXGPRT vector, giving pKO-AMA1. This vector contains the HXGPRT gene (hypoxanthine xanthine guanine phosphoribosyl transferase) for plasmid selection in T. gondii. Vector integration in Δ ku80 genome was verified with PCRs 1 and 2 using the primer pairs ML314/ML673 and ML314/ML393, respectively (see Supplementary Table 2 for primer sequences), and led to the disruption of AMA1 in two non-functional copies. ( b ) IFAs on intracellular Δ ku80 or KO-AMA1 strains using anti-AMA1 ectodomain and anti-MIC3 antibodies. Scale bars, 5 μm. ( c ) Immunoblot carried out on Δ ku80 or KO-AMA1 parasites shows the absence of AMA1 in the mutant using anti-AMA1 antibodies directed against the full ectodomain (domains DI, DII and DIII) and anti-AMA1 tail antibodies. ( d ) Invasion rates of Δ ku80 and KO-AMA1 compared over time during a 5-min invasion assay. Intracellular parasites were scored using a red–green differential antibody staining. Values represent mean±s.e.m ( n =3). ( e ) Left panel: IFAs of KO-AMA1 parasites following invasion assay; red arrow, rhoptry secretion in absence of attached parasite. Scale bar, 5 μm. Right panel: quantification of the abortive invasions in Δ ku80 and KO-AMA1 cell lines. Student’s t -test, ** P <0.05; mean±s.e.m. ( n =3). ( f ) In situ hybridization assay in KO-AMA1 using GST-RON2-2 protein reveals an additional MIC partner for RON2, different from AMA1. Scale bars, 5 μm. ( g ) Invasion rates of KO-AMA1 parasites ±5 μM TgRON2sp. Student’s t -test, * P <0.05; mean±s.e.m. ( n =3). Full size image The genome of T. gondii encodes two AMA1 homologues, TGME49_300130 and TGME49_315730, the latter named sporoAMA1 (ref. 24 ) (or AMA3 in this study, see Supplementary Table 1 for nomenclature) referred to a sporozoite-specific isoform that is able to pair exclusively with a RON2 homologue, namely RON2 L2 (or sporoRON2) [24] . In the KO-AMA1 mutant, we observed a threefold transcriptional upregulation of TGME49_300130 ( Fig. 6a ), named hereafter AMA2 ( Supplementary Table 1 ). This was then confirmed at the protein level in endogenously tagged AMA2 in the parental or the KO-AMA1 background ( Fig. 6b and Supplementary Fig. 4a,b ). Furthermore, we established that AMA2 is a micronemal protein ( Fig. 6c ) that is barely detectable in Δ ku80 line but vastly overexpressed in the KO-AMA1 background ( Supplementary Fig. 4c ). Collectively, these results demonstrate that depletion of AMA1 resulted in the upregulation of AMA2. We then demonstrated that AMA2 is a partner for RON2 by enzyme-linked immunosorbent assay (ELISA) using recombinant AMA2 protein ( Supplementary Fig. 4d ), although the affinity was lower than for generic AMA1 and in vivo by co-immunopurification of AMA2 in the KO-AMA1 line using anti-RON2 antibodies ( Fig. 6d ). Definitive evidence of the functional relevance of AMA2–RON2 interaction for MJ formation and invasion was obtained with the detection of AMA2 at the MJ ( Fig. 6e ) and the knockout of AMA2 in Δ ku80 and KO-AMA1 lines ( Supplementary Fig. 5a,b ). The loss of AMA2 abrogated GST-RON2-2 binding in KO-AMA1 ( Fig. 6f ), thereby establishing that AMA2 is a micronemal partner of RON2. The deletion of AMA2 in KO-AMA1 parasites did not affect replication ( Supplementary Fig. 5c ) but led to a substantial decrease of the residual invasion compared with KO-AMA1 ( Fig. 6g ), indicating that the primary invasion pathway that compensates for the loss of AMA1 relies on AMA2 and its capacity to interact with RON2. Collectively, these data reveal the existence of an alternative pair (AMA2–RON2) allowing T. gondii tachyzoites to invade host cell in a MJ-dependent fashion in the absence of AMA1. 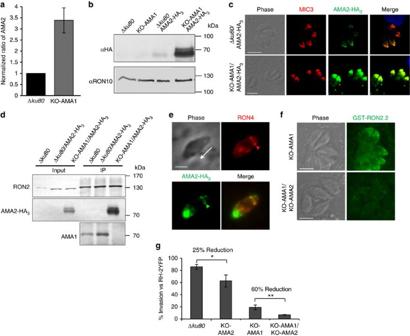Figure 6: A compensatory invasion pathway involves the interaction between AMA2 and RON2. (a) Transcript levels ofAMA2in Δku80or KO-AMA1 line. Values represent the mean±s.d. of three independent experiments. (b) Immunoblot or (c) IFAs of AMA2-HA3in Δku80or KO-AMA1 background. RON10, loading control. MIC3, micronemal marker. Scale bars, 5 μm. (d) Co-immunoprecipitation using anti-RON2-4 antibodies on Δku80/AMA2-HA3or KO-AMA1/AMA2-HA3, followed by an immunoblot revealed with anti-RON2-3 (‘RON2’), anti-HA (‘AMA2-HA3’) or anti-AMA1 (‘AMA1’) antibodies. Δku80strain, negative control. (e) IFA of RON4 and AMA2-HA3in invading KO-AMA1/AMA2-HA3parasites; arrows show the MJ; white arrow, parasite movement. Scale bar, 2 μm. (f)In situhybridization assay using GST-RON2-2 protein on intracellular KO-AMA1 or KO-AMA1/KO-AMA2 mutants. Scale bars, 5 μm. (g) Invasion assay of Δku80, KO-AMA2, KO-AMA1 and KO-AMA1/KO-AMA2 strains performed as described previously20. Student’st-test, **P<0.01; mean±s.e.m. (n=3). Figure 6: A compensatory invasion pathway involves the interaction between AMA2 and RON2. ( a ) Transcript levels of AMA2 in Δ ku80 or KO-AMA1 line. Values represent the mean±s.d. of three independent experiments. ( b ) Immunoblot or ( c ) IFAs of AMA2-HA 3 in Δ ku80 or KO-AMA1 background. RON10, loading control. MIC3, micronemal marker. Scale bars, 5 μm. ( d ) Co-immunoprecipitation using anti-RON2-4 antibodies on Δ ku80 /AMA2-HA 3 or KO-AMA1/AMA2-HA 3 , followed by an immunoblot revealed with anti-RON2-3 (‘RON2’), anti-HA (‘AMA2-HA 3 ’) or anti-AMA1 (‘AMA1’) antibodies. Δ ku80 strain, negative control. ( e ) IFA of RON4 and AMA2-HA 3 in invading KO-AMA1/AMA2-HA 3 parasites; arrows show the MJ; white arrow, parasite movement. Scale bar, 2 μm. ( f ) In situ hybridization assay using GST-RON2-2 protein on intracellular KO-AMA1 or KO-AMA1/KO-AMA2 mutants. Scale bars, 5 μm. ( g ) Invasion assay of Δ ku80 , KO-AMA2, KO-AMA1 and KO-AMA1/KO-AMA2 strains performed as described previously [20] . Student’s t- test, ** P <0.01; mean±s.e.m. ( n =3). Full size image A second AMA–RON pair is upregulated in KO-AMA1 The residual invasion displayed by the double KO-AMA1/KO-AMA2 mutant prompted us to search for additional alternative invasion pathways and specifically to investigate the possible contribution of the second RON2 homologue, RON2 L1 (TGME49_294400). The RON2 L1 gene had two different transcription start sites generating proteins of different sizes, both containing the same C-terminal end, but only the larger one (166 kDa) harbouring a signal peptide allowing its entry in the secretory pathway and subsequent targeting to the secretory organelles ( Supplementary Fig. 6a,b ). As a first step, we endogenously tagged RON2 L1 in the parental or the KO-AMA1 line ( Supplementary Fig. 6c ). Importantly, RON2 L1 was differentially expressed in the two backgrounds ( Fig. 7a ), with an upregulation of the full-length RON2 L1 in KO-AMA1 mutant. RON2 L1 was found both outside the rhoptries and co-localizing with RON2 ( Fig. 7b ), with a labelling in the rhoptry neck more frequently observed in KO-AMA1 mutant. Furthermore, in situ binding and ELISA assays using a fusion protein GST-RON2-2 L1 , which correlates with the RON2-2 region, showed that RON2 L1 recognized a different MIC protein from AMA1, AMA2 ( Fig. 7c ) or AMA3 ( Supplementary Fig. 7 ). The binding was consistently stronger in KO-AMA1 and KO-AMA1/KO-AMA2 mutants compared with parental line, indicating that these mutants upregulated a MIC recognized by RON2 L1 . 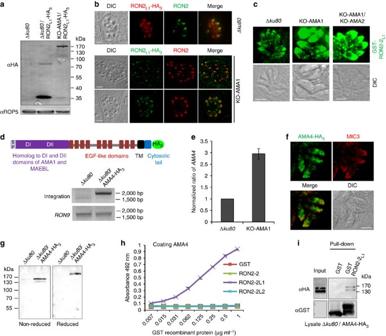Figure 7: A third invasion pathway involves RON2L1and a new MIC protein AMA4. (a) Immunoblot and (b) IFAs of RON2L1-HA3in Δku80or KO-AMA1 background. ROP5, loading control. DIC: Differential Interference Contrast. Scale bars, 5 μm. (c)In situhybridization assay using GST-RON2-2L1protein reveals a micronemal partner for RON2-2L1. GST-RON2-2L1recognized a protein in the micronemes of Δku80parasites as evidenced by the fluorescence detected with anti-GST antibodies. This micronemes labelling was consistently stronger in the KO-AMA1 or KO-AMA1/KO-AMA2 background, suggesting that RON2L1partner was upregulated in absence of AMA1 and did not correspond to AMA2. DIC: Differential Interference Contrast. Scale bars, 5 μm. (d) Upper panel shows a scheme of the predicted domains of AMA4 (SP: signal peptide, TM: transmembrane domain). Lower panel shows the verification of AMA4-HA3tagging in Δku80by PCR. (e) Transcript levels ofAMA4in Δku80or KO-AMA1 line. Values represent the mean±s.d. of three independent experiments. (f) IFA performed on Δku80/AMA4-HA3line localizes AMA4 in the micronemes. DIC: Differential Interference Contrast. Scale bars, 5 μm. (g) Immunoblot of Δku80or Δku80/AMA4-HA3parasites using anti-HA antibodies. (h) ELISA performed with recombinant AMA4_DI-DII-1EGF protein and increasing concentrations of GST-RON2-2, GST-RON2-2L1, GST-RON2-2L2or GST as a control. (i) GST pull-down assay using either GST (as a control) or GST-RON2-2L1and a lysate of Δku80/AMA4-HA3parasites. Immunoblot with anti-GST and anti-HA antibodies. Figure 7: A third invasion pathway involves RON2 L1 and a new MIC protein AMA4. ( a ) Immunoblot and ( b ) IFAs of RON2 L1 -HA 3 in Δ ku80 or KO-AMA1 background. ROP5, loading control. DIC: Differential Interference Contrast. Scale bars, 5 μm. ( c ) In situ hybridization assay using GST-RON2-2 L1 protein reveals a micronemal partner for RON2-2 L1 . GST-RON2-2 L1 recognized a protein in the micronemes of Δ ku80 parasites as evidenced by the fluorescence detected with anti-GST antibodies. This micronemes labelling was consistently stronger in the KO-AMA1 or KO-AMA1/KO-AMA2 background, suggesting that RON2 L1 partner was upregulated in absence of AMA1 and did not correspond to AMA2. DIC: Differential Interference Contrast. Scale bars, 5 μm. ( d ) Upper panel shows a scheme of the predicted domains of AMA4 (SP: signal peptide, TM: transmembrane domain). Lower panel shows the verification of AMA4-HA 3 tagging in Δ ku80 by PCR. ( e ) Transcript levels of AMA4 in Δ ku80 or KO-AMA1 line. Values represent the mean±s.d. of three independent experiments. ( f ) IFA performed on Δ ku80/ AMA4-HA 3 line localizes AMA4 in the micronemes. DIC: Differential Interference Contrast. Scale bars, 5 μm. ( g ) Immunoblot of Δ ku80 or Δ ku80 /AMA4-HA 3 parasites using anti-HA antibodies. ( h ) ELISA performed with recombinant AMA4_DI-DII-1EGF protein and increasing concentrations of GST-RON2-2, GST-RON2-2 L1 , GST-RON2-2 L2 or GST as a control. ( i ) GST pull-down assay using either GST (as a control) or GST-RON2-2 L1 and a lysate of Δ ku80 /AMA4-HA 3 parasites. Immunoblot with anti-GST and anti-HA antibodies. Full size image BLAST analysis using AMA2 and AMA3 as templates retrieved a predicted ORF (open reading frame), TGME49_294330, that harbours in its N-terminus a domain displaying similarities with the DI and DII domains of AMA2 and AMA3, as well as with those of P. falciparum AMA1 and MAEBL (merozoite apical erythrocyte-binding ligand) proteins ( Fig. 7d ). Interestingly, the KO-AMA1 line was shown to overexpress TGME49_294330 by threefold ( Fig. 7e ), which prompted us to verify the expression and localization of the corresponding protein. Endogenous tagging of TGME49_294330 in the Δ ku80 background revealed that it codes for a protein localized to the micronemes ( Fig. 7f,g ), named hereafter AMA4. To establish whether AMA4 acts as a partner for RON2, RON2 L1 or RON2 L2 , we produced a recombinant protein containing DI- and DII-like domains plus a single EGF-like domain (AMA4_DI-DII-1EGF). ELISA using recombinant GST-RON2-2, GST-RON2-2 L1 and GST-RON2-2 L2 proteins showed a direct interaction between GST-RON2-2 L1 and AMA4_DI-DII-1EGF ( Fig. 7h ), which was then confirmed by a pull-down assay using GST-RON2-2 L1 -coupled beads and a lysate of HA-tagged AMA4 parasites ( Fig. 7i ). These results demonstrate that RON2 L1 interacts in a selective and exclusive manner with AMA4, underscoring a third AMA–RON pair to assist invasion in Toxoplasma . The work reported here sheds new light on the recent controversies regarding the precise role of one of the leading erythrocytic stage vaccine candidate, AMA1. Our findings definitively establish that the intimate attachment of the parasite to the host cell, called ‘moving-junction’, results from a cooperation between the parasite proteins RON2 (secreted into the host cell) and AMA1 (displayed on the parasite surface). Moreover, we identify novel AMA–RON pairs that reflect the considerable genetic and molecular plasticity at the disposal of Apicomplexa to compensate for dysfunction in the core invasion machinery. The MJ is a unique structure conserved across the Apicomplexa phylum that is central to the invasion process. A model whereby assembly of the MJ resulting from a cooperation between a complex of parasite Rhoptry Neck proteins including RON2 secreted into the host cell and AMA1 displayed on the parasite surface has been previously proposed [25] . Two recent papers questioned this model [8] , [9] and stated that AMA1 and the RON proteins act independently during parasite invasion, with AMA1 supposedly acting in an earlier attachment/recognition step preceding MJ formation and having no role in parasite internalization into the host. However, those studies did not explore the possibility that alternative mechanisms might compensate for AMA1 dysfunction. Our findings contradict some of the conclusions of the two studies [8] , [9] , and shed new light to reconcile several points of disagreement. We first established by IFA the existence of a bridge between AMA1 and RON2 at the host–cell interface during invasion, and provide direct evidence that an optimal AMA1–RON2 interaction is necessary to withstand the sheering mechanical forces involved in host–cell invasion, a result already suggested by our previous structural analysis [12] , [13] . We then engineered a RON2 mutant specifically impaired in its ability to bind AMA1. Using this KD-RON2 IL/AA mutant, we demonstrated that a decrease in the binding affinity of AMA1–RON2 correlates with a decreased capacity of the parasite to intimately engage the host cell. Parasites lacking either RON2 or AMA1, or a KD-RON2 IL/AA mutant, secrete the contents of the rhoptries, a step that follows the initial attachment of MICs with host receptors, insert the MJ RONs-complex in the host cell membrane, but eventually detach ( Fig. 2b,c and Fig. 3e ). Consequently, the altered intimate attachment observed does not reflect a particular failure in the initial attachment mediated by MICs, but instead argues in favour of a cooperative role of AMA1 and RON2 in structuring the MJ. In the two previous studies [8] , [9] , the authors measured the global attachment defect of conditional or clean KO-AMA1, but did not consider the fact that a failure to establish a firm MJ could also lead to parasite detachment from the host cell. The global altered zoite attachment to host cell observed in those two studies both for Toxoplasma and Plasmodium is therefore compatible with a MJ defect, as evidenced in this work. We next investigated the involvement of AMA1 during the downstream internalization step. We showed that parasites expressing a mutant form of AMA1 within the cytosolic tail were fully competent to secrete the content of the rhoptries and to form a MJ, and as such are intimately attached to the host cell. However, they failed to proceed further and penetrate the host. This demonstrates that AMA1 is not only involved in attachment as recently claimed [8] but also in the internalization step. The MJ is supposed to serve as a point of traction where the parasite pushes entry into the host cell and generates the PVM derived from the invaginated host plasma membrane. An association between the cytoplasmic tail of AMA1 and aldolase [17] , [21] , [26] was previously reported, and proposed to act as a bridge with F-actin and the gliding machinery necessary for internalization. However, a recent report revisiting the implication of aldolase in gliding and invasion [27] showed that aldolase does not have an essential role in coupling AMA1 or other MIC proteins to the actomyosin system during invasion. How the AMA1 tail functions during internalization remains an important question for the future. By scrutinizing the KO-AMA1 line, we provide direct evidence for two alternate pathways that promote assembly of the MJ and hence critically expand the MIC-RON interacting repertoire of T. gondii to four possible complexes composed of AMA1–RON2, AMA2–RON2, AMA3–RON2 L2 (sporo-pair) [24] and AMA4–RON2 L1 ( Fig. 8 ). Therefore, the invading AMA1 mutant parasites display no major changes in MJ architecture because the parasite uses paralogs of the generic AMA1–RON2 pair as substitutes. Hence, our data provide strong support and validation for the current MJ model, based on the cooperation between MIC and rhoptry neck proteins. The labelling of the MJ with a clear RON4- or RON2 ring in AMA1 KO parasites was used as an argument to uncouple AMA1 and RON2 functions [8] , [9] . We clearly demonstrate here the presence of AMA2 at the MJ, its capacity to engage RON2 and hence, the rest of the RONs machinery. Consequently, one can expect to detect the RONs at the MJ, even in absence of AMA1. Concordantly, a strong upregulation of AMA2 transcripts was also observed in the AMA1 KO line in Bargieri et al . [8] Furthermore, similar to what we observe with KO-AMA1 mutant, the AMA1 KO parasites displayed a higher invasion rate compared with the inducible iKO-AMA1 described previously [19] , which also suggests the establishment of a compensatory mechanism during the selection of the parasites. AMA2 overexpression only partially rescues KO-AMA1 invasion. However, we show a weaker affinity of RON2 for AMA2 compared with AMA1 that would explain the sharp decrease in the number of intracellular KO-AMA1 mutant and the concomitant increase in the number of detached parasites. We do not observe an increase in the number of parasites that remain extracellular, stuck onto the host cell via their MJ bridge as shown with mutation in the tail of AMA1 ( Fig. 3 ). All of these results do not point toward a less efficient internalization rate owing to the AMA2 tail but rather indicate a specific defect in structural bridging. According to this hypothesis, the tails of AMA1 and AMA2 are very similar, including the conservation of FW residues. Therefore, once the parasite is correctly anchored to the host cell through alternative AMA–RON pairs, the speed of invasion is not expected to change as reported [8] , [9] . 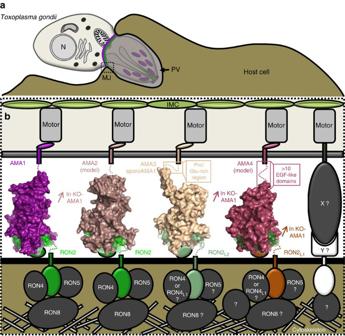Figure 8: Proposed model of theToxoplasmatachyzoite MJ. The model depicts a partially invaded tachyzoite (a) and an enlargement of the MJ (box in dotted lines) in (b). (a) The tachyzoite micronemes and rhoptry necks are coloured in pink and green, respectively. The arrow shows the parasitophorous vacuole (PV), N stands for nucleus. (b) Four AMA–RON interactions bridge the parasite and the host interface, while the cytoplasmic tail of AMA would connect the MJ to the parasite gliding machinery (‘motor’) linked to the inner membrane complex (IMC). The RON4/RON5/RON8 complex, tethered to RON2, localizes beneath the host plasma membrane where it may interact with the host cytoskeleton. The AMA1–RON2 pathway is the main invasion pathway used by the tachyzoite (12and this study) or the merozoite ofPlasmodium13. Three additional invasion routes are used byToxoplasmaand depend on divergent AMA1 and RON2 homologues: (i) AMA2 (homology model) that connects RON2; (ii) AMA3–RON2L2; and (iii) RON2L1that bridges a more distantly-related AMA1 homologue named AMA4 (homology model). The last two pairs are highly expressed during sporozoite stage. Importantly, AMA2–RON2 and AMA4–RON2L1pathways are strongly upregulated in KO-AMA1 tachyzoites, demonstrating a significant molecular plasticity of the MJ to compensate for the loss of AMA1. In addition, yet unidentified, much more divergent components (here named X/Y) might add to the architecture of the MJ. Figure 8: Proposed model of the Toxoplasma tachyzoite MJ. The model depicts a partially invaded tachyzoite ( a ) and an enlargement of the MJ (box in dotted lines) in ( b ). ( a ) The tachyzoite micronemes and rhoptry necks are coloured in pink and green, respectively. The arrow shows the parasitophorous vacuole (PV), N stands for nucleus. ( b ) Four AMA–RON interactions bridge the parasite and the host interface, while the cytoplasmic tail of AMA would connect the MJ to the parasite gliding machinery (‘motor’) linked to the inner membrane complex (IMC). The RON4/RON5/RON8 complex, tethered to RON2, localizes beneath the host plasma membrane where it may interact with the host cytoskeleton. The AMA1–RON2 pathway is the main invasion pathway used by the tachyzoite ( [12] and this study) or the merozoite of Plasmodium [13] . Three additional invasion routes are used by Toxoplasma and depend on divergent AMA1 and RON2 homologues: (i) AMA2 (homology model) that connects RON2; (ii) AMA3–RON2 L2 ; and (iii) RON2 L1 that bridges a more distantly-related AMA1 homologue named AMA4 (homology model). The last two pairs are highly expressed during sporozoite stage. Importantly, AMA2–RON2 and AMA4–RON2 L1 pathways are strongly upregulated in KO-AMA1 tachyzoites, demonstrating a significant molecular plasticity of the MJ to compensate for the loss of AMA1. In addition, yet unidentified, much more divergent components (here named X/Y) might add to the architecture of the MJ. Full size image AMA4–RON2 L1 pair is the most divergent AMA–RON complex and is predominantly expressed at the sporozoite stage according to ToxoDB. This highlights a possible greater diversity of the MJ components along the life-cycle stages of apicomplexan parasites. Interestingly, the protein MAEBL is highly conserved throughout the Plasmodium species, and importantly contains an N-terminal with homology to domains I and II of AMA1. MAEBL is expressed in both midgut and salivary gland sporozoite stages and has an essential role in attachment of the sporozoite to the salivary gland [28] , as well as in sporozoite penetration and development in primary hepatocytes [29] . Thus, MAEBL is a plausible actor during sporozoite invasion of hepatocytes and a potential compensatory molecule in P. berghei AMA1 KO merozoite [8] . Further investigations will be required to determine whether MAEBL can engage a RON protein and thereby contribute to MJ formation. The alternative AMA–RON complexes deployed in absence of AMA1 only partially restore the invasion defect, establishing the generic AMA1–RON2 pair as the central player of tachyzoite invasion. Since RON2 is the common denominator for AMA1 and AMA2, one might expect an upregulated expression of RON2 paralogs in the KD-RON2 strain. However, we did not observe an increased invasion rate of KD-RON2 in continuous culture, in contrast to KO-AMA1. One possible explanation is that the KD-RON2 mutant is not only defective for RON2 but also for RON4 and RON5, the latter being also crucial for invasion [30] . In consequence, a KD-RON2 mutant needs to compensate simultaneously for the loss of three proteins. As there are no RON5 homologues in Toxoplasma genome, a compensatory mechanism for the loss of RON5 might not be possible. This would explain why we failed to obtain a KO-RON2 by the disruption strategy used for AMA1 and argue in favour of the production of minute amounts of RON2, RON4 and RON5 in the KD-RON2 line sufficient to support the 10% residual invasion observed in this strain. Further investigation will be required to determine whether the KD-RON2 mutant has developed alternative pathways to compensate for RON2 dysfunction. Our results uncover additional ligand/receptor molecules forming the MJ that follow the MIC/RON couple paradigm exemplified by AMA1/RON2 and hence reveal a much broader repertoire of junctional proteins available to the apicomplexan parasites. This study also highlights the ability of these resourceful and versatile parasites to compensate for deleterious mutations through an intriguing reliance on molecular plasticity, which might also apply in other key events of the life cycle in Apicomplexa. Ethics statement This study was conducted according to the European Union guidelines for the handling of laboratory animals, and the immunization protocol for antibody production in rabbits was conducted at the CRBM animal house (Montpellier) and approved by the Committee on the Ethics of Animal Experiments (Languedoc-Roussillon, Montpellier; permit number: D34-172-4, delivered on 20/09/2009). Parasite cultures All T. gondii tachyzoites were passaged in human foreskin fibroblasts (HFFs) (American Type Culture Collection-CRL 1634) or Vero cells (American Type Culture Collection CCL 81) grown in Dulbecco’s modified essential medium (Gibco-BRL) supplemented with 10% fetal calf serum and 2 mM glutamine. Tachyzoites of the T. gondii RH strain deleted for ku80 gene (Δ ku80 ) [31] were used throughout the study. Invasion assays Except when noted in figure legends, the invasion was performed as follows. Freshly released tachyzoites (5 × 10 6 ) were incubated 20 min at 4 °C on confluent HFFs grown on coverslips in 24-well plates. Invasion was allowed to take place during 5 min at 38 °C before fixation with 4% paraformaldehyde for 30 min at room temperature. A dual-labelling screen with anti-SAG1 (ref. 32 ) (dilution 1:1,000) and anti-ROP1 (ref. 5 ) (dilution 1:1,000) antibodies was used to discriminate between extracellular versus intracellular parasites. Intracellular parasites were determined by microscopic examination of at least 30 fields per coverslip ( n =3 coverslips). Independent invasion assays were performed at least three times. Inhibitions of invasion were carried out using parasites pre-incubated for 20 min at 4 °C with 5 μM of Tg RON2sp [12] before proceeding to 5 min invasion. Alternatively, invasion assays were performed upon co-inoculation of wild-type (RH-2YFP) used as an internal control and the strain to be tested, as described previously [20] . Quantification of abortive invasion To quantify the number of abortive invasion, IFA after 5 min invasion (see invasion) was performed with anti-RON4 (ref. 33 ) (mouse monoclonal antibodies MAb T54H1, undiluted hybridoma culture supernatant) and anti-ROP1 (ref. 5 ) (dilution 1:1,000), and the number of dual ROP1/RON4 staining in absence of detectable parasite by phase contrast was determined. Alternatively, 5 × 10 5 parasites were added to confluent HFFs monolayer for 2 h at 37 °C, then extensively washed with Hank’s Balanced Salt Solution to remove extracellular parasites. IFA was performed 20 h later using anti-phospho-Stat6 (dilution 1:100; Cell Signaling Technology Inc.) and anti-ROP2-3-4 (ref. 34 ) antibodies (dilution 1:100) to label the host nuclei and the parasite vacuoles respectively. P-STAT6 + cells containing a vacuole (productive invasions) or not (abortive invasion) were determined by microscopic examination of at least 30 fields per coverslip ( n =3 coverslips). Two independent experiments have been performed. Preparation of T. gondii genomic DNA and RNA Genomic DNAs were prepared from tachyzoites using the Wizard SV genomic DNA purification system (Promega). RNA was isolated from tachyzoites using Nucleospin RNA II Kit (Macherey-Nagel), cDNA was produced by reverse transcription (RT-PCR) with the Superscript First-Strand Synthesis System for RT-PCR (Invitrogen) according to the manufacturer’s instructions. Quantitative PCR Total RNA was extracted and purified using the NucleoSpin RNAII kit (Macherey-Nagel). Extraction method was validated using an Agilent Bioanalyser 2100 with Agilent RNA 6000 Nano Kit. RNA Integrity Number ≥9 was obtained consistently. cDNA preparations were obtained by reverse transcription using Superscript III First-Strand Synthesis SuperMix for quantitative RT-PCR (qRT-PCR; Invitrogen) and 800 ng of total RNA. All specific primers used for qPCR experiments are listed in the Supplementary Table 2 . qPCR were carried out using 1 μM of each primer, Roche Light-Cycler 480 SYBR Green I Master and cDNA in 6 μl reaction mixture. Forty five cycles of denaturation (10 s, 95 °C), annealing (10 s, 60 °C) and elongation (10 s, 72 °C) were performed on a Light Cycler 480 Instrument. On amplification curves, we rejected Cq>38 and on fusion curves we retained single peak only. Relative quantification was performed by Light Cycler 1.5 Software according to Michael W. Pfafll Model [35] . To normalize the results, actin was selected as a reference gene (variability of actin expression between different mutants was <1Cq). Cloning of DNA constructs All the PCR amplifications were performed with either La Taq (TaKaRa) or the Phusion polymerases (NEB Biolabs), and the primers are listed in the Supplementary Table 2 . Plasmid pKD-TgRON2 was designed to produce KD-RON2 line. It is based on plasmid pTUB8TATi-1-HX-TetO7-SAG1 (ref. 36 ) (a gift from Drs Daher and Soldati-Favre), which contains a transactivator (TATi) promoting transcription of genes placed under the modified SAG1 promoter, TetO7-SAG1, encompassing several TetO sequences. Addition of ATc in the medium prevents the binding of TATi to the TetO sequences and therefore precludes transcriptional activation of the gene of interest. The HXGPRT gene (hypoxanthine xanthine guanine phosphoribosyl transferase) encodes a genetic marker suitable for T. gondii -positive selection. The pTUB8TATi-1-HX-TetO7-SAG1 plasmid has been modified to replace the native RON2 promoter with an ATc-repressible SAG1 promoter. To this end, 1 kb of the RON2 5′UTR was amplified by two distinct PCRs using the couples of primers ML772/ML773 and ML774/ML775. The 5′UTR was then cloned NcoI/StuI upstream of the TATi-1 sequence. Similarly, 1 kb of the RON2 5′coding sequence was amplified with primers ML936 and ML937, and was cloned AvrII/SpeI downstream of the TetO7-SAG1 promoter. pKD-TgRON2 was digested with SbfI to allow genomic integration by double-homologous recombination. To complement the KD-RON2 line with a wild-type or mutated copy of RON2 , we used a modified version of pUPRT-TUB-G13-Ty plasmid that allows vector integration at the UPRT locus [37] . First, an ApaI restriction site was added downstream of the 3′UPRT by site-directed mutagenesis using primers ML1214 and ML1215. Then, the tubulin promoter was replaced in BglII/NotI by a 1.5-kb fragment of the RON2 5′UTR amplified with primers ML1216 and ML1217. Finally, a wild-type version of the RON2 cDNA amplified with primers ML1218 and ML1219 or a mutated version for residues I1318-L1319 (IL/AA) was introduced in Pac I/ Eco RV in place of the G13 gene. Mutagenesis of the RON2 cDNA was performed using primers ML728 and ML729. The resulting vectors, named pcKD-TgRON2-WT and pcKD-TgRON2-IL/AA, respectively, were linearized with Apa I before transfection. Disruption of AMA1 gene was performed using the plasmid pKO-AMA1, derived from the p3Ty-HXGPRT vector [38] in the following manner. An internal AMA1 fragment was PCR amplified using the couple of primers ML883/ML884, and subsequently cloned in the p3Ty-HXGPRT using the restriction sites Kpn I and Nsi I. pKO-AMA1 was linearized with PstI before transfection. The HA 3 -tagging at the endogenous locus of AMA2, RON2 L1 and AMA4 was performed by inserting the C-terminal part of the corresponding genes in frame with the HA 3 tag in the vector pLIC-HA 3 -DHFR using the ligation-independent-cloning strategy [31] . The C-ter parts of RON2 L1 and AMA4 were PCR amplified using the couples of primers ML813/ML814 and ML1461/ML1462, respectively. For AMA2 , a unique Nco I site was introduced by amplification of two distinct PCR fragments using the couples of primers ML1518/ML1596 and ML1597/ML1521 that were ligated before insertion in pLIC-HA 3 -DHFR. The resulting vectors pLIC-AMA2-HA 3 -DHFR, pLIC-RON2 L1 -HA 3 -DHFR and pLIC-AMA4-HA 3 -DHFR were linearized with Nco I, Nco I and Apa I, respectively, before transfection to allow single homologous recombination. To generate the knockout vector pKO-AMA2, 2.2 kb of both the 5′UTR and 3′UTR of AMA2 gene (ToxoDB accession no. TGME49_300130) were amplified from genomic DNA and cloned into the p2854-TgDHFR vector (see Supplementary Table 2 for primers). Δ ku80 parasites were transfected with 40 μg of the pKO-AMA2 vector linearized with Not I/ Nsi I to allow gene replacement by double-homologous recombination. Parasites resistant to pyrimethamine were isolated by limiting dilution cloning and were subsequently screened by PCR for the loss of AMA2 gene using primers listed in the SI. Plasmid pGEX-TgRON2-2 was described in Lamarque et al. [6] Plasmids pGEX-TgRON2-2 L1 and pGEX-TgRON2-2 L2 were designed to express a N-terminal GST-tagged recombinant RON2-2 L1 or RON2-2 L2 protein that corresponds to the RON2-2 domain of RON2 (Q1284 to A1330 for RON2-2 L1 and I453 to G503 for RON2-2 L2 ). The corresponding fragments were amplified from cDNA with primers ML817/ML818 and ML819/ML820, respectively. Production of recombinant proteins and serum GST-tagged proteins were produced as described previously [6] and were purified by affinity purification on gluthatione–agarose column in native conditions according to the manufacturer’s instructions. Recombinant proteins were dialysed against PBS pH 7, concentrated on Amicon Ultra 3K and quantified by Pierce BCA protein assay. Recombinant TgRON8 was used to produce anti-RON8n antibodies ( Supplementary Fig. 8 ). A PCR product corresponding to amino acids 65–532 of RON8 was amplified from T. gondii tachyzoites cDNA, with primers ML162 and ML163. It was then cloned into pGEX-4T-3 (GE Healthcare) and the construct was transformed into Escherichia coli C41 cells to produce a recombinant protein with a N-terminal glutathione-S transferase tag, which is used to immunize a rat. Recombinant His-tagged AMA1 and sporoAMA1 proteins were produced in baculovirus [12] , [24] . His-tagged AMA1 was used to immunize rabbits and produce polyclonal antibodies (anti-AMA1 S48) as described previously [5] . For recombinant AMA4, a sequence encoding the region of TgAMA4 that aligns with DI and DII of Toxoplasma generic AMA1 and the first EGF domain (TgAMA4_DI-DII-1EGF) was amplified out of the full-length sequence that was codon optimized for insect cells and synthesized by GenScript. A sequence encoding the region of AMA2 that aligns with the complete DI, DII and DIII ectodomain of Toxoplasma generic AMA1 (AMA2_ecto) was codon optimized for insect cells and synthesized by GenScript. Both sequences were cloned into a modified pAcGP67b vector (Pharmingen) incorporating a C-terminal hexahistidine tag separated from the protein of interest by either a thrombin or TEV cleavage site. Viruses encoding TgAMA4_DI-DII-1EGF and AMA2_ecto for insect cell expression were generated and amplified according to established protocols [12] . For large-scale expression, Hi5 cells in ESF-921 (Expression Systems LLC, USA) or Lonza (VWR, Canada) were infected with high titre virus for 65 h, after which time the supernatant was harvested and concentrated, and the target proteins were purified by nickel affinity chromatography. The hexahistidine tag was removed, and the samples were further purified by size exclusion chromatography (Superdex 16/60 75 or 200) in HEPES buffered saline. The final yields of TgAMA4_DI-DII-1EGF and AMA2 were 14 and 0.3 mg, respectively, of purified protein per litre of insect cell culture. cDNA annotations and 5′RACE Amplification of TgAMA2 and TgRON2 L 1 cDNAs was done by PCR with primers ML824/ML1525 and ML827/ML814, respectively. These PCR fragments were cloned in the TOPO Zero Blunt vector (Invitrogen) and sequenced (Eurofins MWG operon). 5′RACE was used to characterize the 5′ ends of TgRON2 L1 using 5′RACE system for Rapid Amplification of cDNA Ends Version 2.0 (Invitrogen) according to the manufacturer’s instructions. First-strand cDNA synthesis was obtained using ML1654 as gene-specific reverse primer. Then, homopolymeric tails (dC) were added to the cDNA 3′ ends. This extension allows the hybridization of the forward Abridged Anchor Primer. Finally, PCR was performed using Abridged Anchor Primer and ML1655. As no amplification was detected, two subsequent nested PCRs were done using ML1656 then ML1607 as reverse primers. A detectable amplification (~1,300 bp) was obtained and cloned in the TOPO Zero Blunt vector (Invitrogen) for sequencing with SP6 and M13. Transfection and selection of transformants 15 × 10 6 T. gondii tachyzoïtes were transfected by electroporation at 2.02 kV, 50 Ω and 25 μF in a Electro Cell Manipulator 630 (BTX) with 30–50 μg plasmid DNA. All the plasmids used were linearized prior transfection. The transgenic parasites were selected by addition of pyrimethamine at 2 μM for the pLIC-HA 3 -DHFR-derived vectors and pKO-AMA2; mycophenolic acid at 25 μg ml −1 plus xanthine at 50 μg ml −1 for pKD-TgRON2 and pKO-AMA1 vectors; and FUDR at 5 μM for pcKD-RON2 WT and IL/AA. For each transfection, clones were isolated by limiting dilution cloning and screened by PCR for correct vector integration. Plaque assay and intracellular replication For plaque assay, confluent monolayers of HFFs grown in six-well plates were infected with ~50 tachyzoites per well and incubated for 6–7 days at 37 °C. They were then fixed in cold methanol for 20 min and stained with Giemsa. Images were obtained with an Olympus MVX10 macro zoom microscope equipped with an Olympus XC50 camera. Plaque area measurements were performed with Cell A software (Olympus). For intracellular growth assay, confluent monolayers of HFFs were infected with 2 × 10 5 freshly released tachyzoites. Two hours post infection, HFFs cells were washed three times with Hank’s Balanced Salt Solution (Gibco-BRL) to remove extracellular parasites and fixed 20 h later with 4% paraformaldehyde for staining with anti-SAG1. The number of parasites per vacuole were counted for 200 vacuoles per coverslip, done in triplicate. The experiments have been carried out three times. Immunofluorescence microscopy IFA of infected monolayers of HFFs cells were conducted as described previously [5] . The antibodies used and their dilution for IFA are listed in Supplementary Table 3 . Images were acquired either with a Leica DMRA2 microscope equipped for epifluorescence, the images being recorded with a COOLSNAP CCD camera (Photometrics) driven by the Metaview software (Universal Imaging Co.) or with a Zeiss Axioimager epifluorescence microscope and images were recorded with a Zeiss Axiocam MRm CCD camera driven by the Axiovision software (Zeiss) at the Montpellier RIO imaging facility. Pull-down, co-immunoprecipitation and ELISA Parasite solubilization in 1% NP40 and immunosorption procedures [33] were done using rabbit anti-TgAMA1 (ref. 6 ) (anti-unfolded ectodomain I, II and III; dilution 1:1,000), anti-RON2-4 (ref. 6 ) (dilution 1:1,000) or anti-HA antibodies (rat MAb anti-HA (Roche, clone 3F10), dilution 1:100). For GST pull-down experiments, 0.5 μM of GST or GST-RON2-2 L1 recombinant proteins were bound to Glutathione-agarose beads. Lysates from 400 × 10 6 extracellular parasites were incubated overnight with the corresponding beads. Washes were performed twice in wash buffer 1 (50 mM Tris pH 8.0, 150 mM NaCl, 4 mM EDTA and 1% NP40) and once in wash buffer 2 (5 mM Tris pH 6.8) as described in Lamarque et al. [6] Elution from beads was performed during 5 min at 95 °C with SDS-PAGE sample buffer. Western blots were performed on the eluates using anti-RON2-3, rabbit anti-TgAMA1 or anti-HA antibodies. The antibody dilutions used for western blot are described in Supplementary Table 3 . Full size blots can be found in Supplementary Fig. 9 . ELISAs were performed as described previously [6] . Tg AMA2- Tg RON2D3 and Tg AMA4- Tg RON2 L1 D3 homology modelling The core structural model for Tg AMA2 (Ser45 to Asn467; TGME49_300130) was initially generated using the iTASSER server [39] based off Tg AMA1 chain A of the Tg AMA1- Tg RON2sp co-structure (PDB ID 2Y8T), with which it shares 32% identity. Apical surface loops were removed and multiple conformations were generated for loops other than the DII loop (Thr327 to Lys356) using Modeller 9v8 through the Chimera interface [40] , [41] ; the final model of Tg AMA2 was chosen based on a combination of its low value of the normalized Discrete Optimized Protein Energy value (zDOPE) and orientations of apical loops not blocking access to the central groove. The coordinates for the core 30 residues (Gln1300 to Ala1329; TGME49_300100) of Tg RON2, named hereafter Tg RON2D3, were taken from the co-structure with Tg AMA1, and initially docked into the Tg AMA2 groove using ProtInfoPPC [42] . The Tg AMA2- Tg RON2D3 model was refined using Rosetta FlexPepDock [43] with the complex showing the lowest Rosetta energy score chosen and validated by visual inspection, PISA [44] , ProQ [45] , ERRAT [46] and MolProbity [47] . Tg AMA4 shows an average of 21% identity with the three other Tg AMAs, and with an ectodomain of ~1,000 amino acids, it is also more than twice the size, whereas the DI-like/DII region of Tg AMA4 still has only 21% identity with Tg AMA1 DI/DII, it is just 25% larger. The iTASSER server [39] was used to generate a model of Tg AMA4 DI-like/DII (Ser31 to Leu491; TGME49_294330) based on a number of characterized apicomplexan AMA structures. A high-confidence model for the core region could be identified based on disulphide connectivity, but extensive loop insertions containing cysteines with unknown disulphide bonding patterns limited the ability to generate an overall high-confidence model of Tg AMA4. All of the models showed the possibility for a groove in the apical surface of Tg AMA4, so the model with the highest confidence score was chosen and the apical loops were trimmed to expose the groove. A model of Tg RON2 L1 D3 (Qln1284 to Ser1324; TGME49_294400) generated by mutation of Tg RON2sp was manually docked into the groove. A crystallized co-structure of Tg AMA4- Tg RON2 L1 D3 will likely show significant differences from the preliminary model presented here, but the overall binding paradigm is expected to be conserved. How to cite this article: Lamarque, M. H. et al. Plasticity and redundancy among AMA–RON pairs ensure host cell entry of Toxoplasma parasites. Nat. Commun. 5:4098 doi: 10.1038/ncomms5098 (2014).